Deep-tissue focal fluorescence imaging with digitally time-reversed ultrasound-encoded light Fluorescence imaging is one of the most important research tools in biomedical sciences. However, scattering of light severely impedes imaging of thick biological samples beyond the ballistic regime. Here we directly show focusing and high-resolution fluorescence imaging deep inside biological tissues by digitally time-reversing ultrasound-tagged light with high optical gain (~5×10 5 ). We confirm the presence of a time-reversed optical focus along with a diffuse background—a corollary of partial phase conjugation—and develop an approach for dynamic background cancellation. To illustrate the potential of our method, we image complex fluorescent objects and tumour microtissues at an unprecedented depth of 2.5 mm in biological tissues at a lateral resolution of 36 μm×52 μm and an axial resolution of 657 μm. Our results set the stage for a range of deep-tissue imaging applications in biomedical research and medical diagnostics. Realizing high-resolution fluorescence imaging within scattering biological tissues is a central goal in biomedical imaging. Considerable efforts have been made to extend the imaging depth of optical methods [1] , [2] , [3] , [4] , [5] , [6] , [7] , but focal excitation of fluorescence has so far been fundamentally limited to a depth of one transport mean free path, or approximately 1 mm in most biological samples. This is because conventional focusing approaches treat scattered light as noise and select for the ballistic light component, which exponentially decreases with depth. However, scattered light contains important information about the sample, which can in fact be utilized. When light passes through scattering samples, its wavefront is seemingly randomized, but the randomization occurs in a deterministic and time-symmetric way. These properties of elastic light scattering have recently been used to focus light through turbid samples by iterative wavefront optimization [8] , [9] , [10] , [11] , [12] , [13] , [14] and by time reversal using optical phase conjugation [10] , [15] , [16] , [17] . These methods are, in many ways, analogous to adaptive optics methods used in astronomy to cancel out the effect of atmospheric scattering [18] , [19] . However, in contrast to astronomy, where it is sufficient to image through a turbid medium (the atmosphere), the goal of biomedical imaging is to image inside. To achieve focusing inside tissues, Xu et al . [20] proposed a scheme termed time reversal of ultrasound-encoded light (TRUE), which combines optical phase conjugation [21] with ultrasound encoding [22] . They used focused ultrasound, which is much less scattered than light in biological tissues, to create a virtual source of light frequency shifted by the acousto-optic effect. Scattered light emanating from this source was then time reversed by a photorefractive crystal acting as a phase conjugate mirror. The authors inferred the formation of a time-reversed optical focus from a line-scan across millimeter-scale absorbers embedded in tissue-mimicking phantoms. Although it promises improved absorption contrast [20] , [23] , [24] , the use of this technique for high-resolution fluorescence imaging in biological tissues remains fundamentally challenging. Because of the low ultrasound modulation efficiency [25] , the phase conjugate mirror has to provide orders of magnitude higher than unity gain to excite detectable fluorescence. This requirement cannot be met by traditional phase conjugate mirrors based on photorefractive crystals, whose gain is typically much less than one [26] , [27] . Moreover, the significant challenge of undesired background illumination because of partial phase conjugation needs to be addressed. With complete time reversal, the TRUE focusing technique can be conceptually represented as photons retracing their paths back to the location of the virtual source. However, this view disregards the wave nature of light: complete time reversal requires full control over phase, amplitude and polarization of the entire scattered field over the full solid angle—which is fundamentally unfeasible (see below). As a result, even with perfectly aligned optics and noise-free recording of the scattered wavefront, the time-reversed focus is necessarily accompanied by a background [28] , [29] , [30] , which would obscure the fluorescence signal originating at the desired optical focus. Here we present a new strategy to overcome these challenges by combining digital phase conjugation [31] with dynamic wavefront manipulation. We directly visualize the formation of an optical focus, exciting fluorescence between layers of highly scattering tissue. In doing so, we confirm the presence of the accompanying background predicted by theory that can be dynamically reproduced and subtracted. This digital background cancellation procedure, along with the high phase conjugate gain and resolution of our technique, enables the first demonstration of focused fluorescence imaging 2.5 mm deep inside biological tissue. Principles Our setup for fluorescence imaging with time-reversed light is diagrammatically shown in Fig. 1 . As the performance of our approach critically depends on achievable resolution, phase conjugate mirror gain and fidelity of phase conjugation, these parameters deserve further discussion. 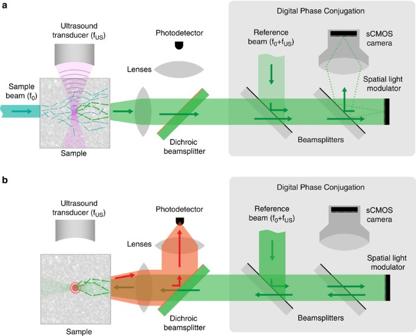Figure 1: Schematic of the imaging principle. (a) In the recording step, a 0.8-mm wide sample beam (f0) scatters as it propagates through the tissue sample. A confined region of the scattered light in the tissue sample is frequency-shifted (f0±fUS) by a focused ultrasound pulse. The ultrasound focus thus becomes a virtual source within the tissue. Both the frequency-shifted light and the non-shifted light further scatter through the tissue and are collected. This output wavefront interferes with a reference beam (f0+fUS) and the resulting interference pattern is imaged onto a scientific CMOS (sCMOS) camera in the digital phase conjugate mirror module. The digital phase conjugate mirror selectively measures the phase map (φ(x,y)) of the frequency-shifted light through digital phase-shifting holography. The ultrasound is turned off after recording. (b) In the playback step, the conjugate of the recorded phase map (−Φ(x,y)) is displayed on a spatial light modulator (SLM) placed at the image plane of the sCMOS camera. The reference beam reflects off the SLM and is transformed into the phase conjugate beam that is propagated back into the tissue, reconstructing an optical focus at the ultrasound modulation location. Any excited fluorescence is collected and measured outside the tissue using a photodetector. Figure 1: Schematic of the imaging principle. ( a ) In the recording step, a 0.8-mm wide sample beam ( f 0 ) scatters as it propagates through the tissue sample. A confined region of the scattered light in the tissue sample is frequency-shifted ( f 0 ± f US ) by a focused ultrasound pulse. The ultrasound focus thus becomes a virtual source within the tissue. Both the frequency-shifted light and the non-shifted light further scatter through the tissue and are collected. This output wavefront interferes with a reference beam ( f 0 + f US ) and the resulting interference pattern is imaged onto a scientific CMOS (sCMOS) camera in the digital phase conjugate mirror module. The digital phase conjugate mirror selectively measures the phase map (φ (x , y )) of the frequency-shifted light through digital phase-shifting holography. The ultrasound is turned off after recording. ( b ) In the playback step, the conjugate of the recorded phase map (−Φ (x , y )) is displayed on a spatial light modulator (SLM) placed at the image plane of the sCMOS camera. The reference beam reflects off the SLM and is transformed into the phase conjugate beam that is propagated back into the tissue, reconstructing an optical focus at the ultrasound modulation location. Any excited fluorescence is collected and measured outside the tissue using a photodetector. Full size image Light scatters as it propagates through tissue, resulting in a speckled light field at the ultrasound focus. The speckles within the ultrasound focus are frequency-shifted by the acousto-optic effect, creating a source of frequency-shifted light ( Fig. 1a ). As our technique selectively records and phase-conjugates the frequency-shifted light, the size of the ultrasound-modulated volume determines the resolution of the phase-conjugated optical focus. We use a high-numerical aperture-focused ultrasound transducer with a calculated focal width of 34 μm. To further confine the ultrasound-modulated volume along the axis of ultrasound propagation, we operate both the ultrasound source and the laser in pulsed mode [32] such that light only enters the sample when the ultrasound pulse has reached the target modulation volume (see Methods ; calculated resolution along the axis of ultrasound propagation: 54 μm). With traditional phase conjugate mirrors, the power in the phase-conjugated beam ( P OPC ) is proportional to the power in the signal beam ( P S ) (ref. 27 ). This proportionality is referred to as the gain of the phase conjugate mirror: Because of the low ultrasound modulation efficiency and the small area ratio between ultrasound focus and scattered wavefront, the scattered light field reaching the phase conjugate mirror consists mostly of light that is not frequency-shifted ( f 0 ) and a minute fraction (in our setup on the order of 10 −4 of the total power) of frequency-shifted, ultrasound-tagged light ( f 0 ± f US ). Therefore, to excite detectable fluorescence at the optical phase conjugate focus, a phase conjugate mirror with gain orders of magnitude larger than unity is required. This is currently not achievable by traditional phase conjugate mirrors, even with advanced phase conjugation schemes [33] , [34] , [35] . To selectively phase-conjugate only the frequency-shifted light with high gain, we implement an improved digital optical phase conjugation scheme (DOPC) that consists of a high dynamic range scientific CMOS (sCMOS) camera and a high-resolution phase-only spatial light modulator (SLM) [31] . The scattered, ultrasound-tagged light field interferes with an equally frequency-shifted reference beam ( f 0 + f US ) and is imaged onto the sCMOS camera. Using digital phase-shifting holography [36] , the phase of the frequency-shifted wavefront (Φ( x , y )) with respect to the reference beam is measured. By reflecting off a phase-only SLM displaying a phase conjugate map (−Φ( x , y )) at the image plane of the camera, the same reference beam is modulated to become a phase conjugate beam that is sent back into the sample ( Fig. 1b ). The phase conjugate beam traverses back through the tissue sample to converge at the location of the ultrasound focus resulting in an optical focus deep inside the tissue sample. In our DOPC setup, the power in the phase conjugate light that leaves the DOPC setup is only dependent on the power in the reference beam that reflects off the SLM displaying the phase conjugate map; thus, the DOPC is fundamentally not limited in terms of gain (equation (1)). In our experiments, we adjusted the intensity of the reference beam during playback to achieve a gain of approximately 5×10 5 , such that the phase conjugate focus contains sufficient energy to excite fluorescence that can be collected and detected outside of the tissue by a photomultiplier tube (PMT). Theoretically, with complete phase conjugation, the light field within the ultrasound focus can be reconstructed without error (see Supplementary Methods ). However, the assumption of complete phase conjugation breaks down in practice—real phase conjugate mirrors, whether based on photorefractive crystals or SLMs, have finite etendue and can only intercept a fraction of the output wavefront. As a result, a background always exists in the case of partial phase conjugation [28] , [29] , [30] . In a random scattering medium, the ratio of the peak intensity of the phase conjugate focus to the average intensity of the accompanying background, the peak-to-background ratio, can be analytically derived. Following the framework of Vellekoop et al . [37] , [38] , we find that the peak-to-background ratio is determined by the number of optical modes intercepted and time-reversed by the phase conjugate mirror, N , and the number of input modes in the ultrasound focus, M (see Supplementary Methods ). When both phase and amplitude of the scattered field are time-reversed, a case similar to the use of traditional phase conjugate mirrors, the peak-to-background ratio is: When only the phase of the scattered field is time-reversed, a case similar to our technique using the DOPC, the peak-to-background ratio for large N is: As N is finite in a real-phase conjugation setup, a phase conjugate background is inevitable. In our experimental setup, N is limited by the number of optical modes imaged onto the SLM and the fact that only the horizontally-polarized component is measured and time-reversed. The diffuse background that inevitably results can excite fluorophores outside of the focus, contributing to noise in the detected fluorescence signal. Because of its spatial extent, the total background excitation can drown out the desired focal fluorescence signal detected by a single channel PMT outside the sample. We show in our experiments that this background, though indeed significant, can be dynamically subtracted by digital manipulation of the measured phase conjugate map, allowing us to realize high-resolution focal fluorescence imaging in biological tissues. Direct visualization of optical focus To directly visualize and characterize the focus formed by time-reversed light, we placed an optically transparent hydrogel slab containing a thin quantum dot layer between two pieces of ex vivo chicken breast tissue, each 2.5 mm thick ( Fig. 2a ). When we focused light into the tissue without any wavefront manipulation (flat phase display on the SLM), the light was highly scattered and failed to form a focus ( Fig. 2b ). In contrast, Fig. 2c shows the fluorescence excited by phase conjugation of ultrasound frequency-shifted light. A cone of light converging into the location of the ultrasound focus was clearly visible, albeit on a significant background. Taking into account the thickness of the quantum dot sheet (500 μm) and the expected size of the ultrasound focus (34 μm, see Methods ), the peak-to-background ratio was determined as ~5.5. 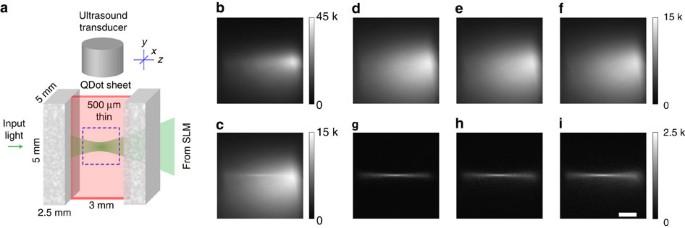Figure 2: Demonstration of optical focusing between thick layers of biological tissue. (a) Schematic of the sample arrangement, consisting of a thin sheet of quantum dots between two 2.5 mm thick sections ofex vivochicken tissue. (b–d) Fluorescence emission camera images of the area (in they–zplane) indicated by the dashed blue square ina. (b) Diffuse illumination pattern obtained by focusing into the tissue without wavefront modulation (flat phase display on the SLM). (c) Illumination pattern resulting from optical phase conjugation of ultrasound-tagged light, showing a focus on top of a diffuse background. (d–f) Background images and (g–i) corresponding background subtracted maps (positive values) obtained by the following techniques: (d,g) mechanically shifting the sample by 5 μm to disrupt phase conjugation; (d,h) digitally shifting the phase map by 50 pixels; and (f,i) modulating the original phase map by subdividing it into 8×16 areas and alternately adding 0 or π phase shift to each area (seeMethods). Scale bar, 500 μm. Figure 2: Demonstration of optical focusing between thick layers of biological tissue. ( a ) Schematic of the sample arrangement, consisting of a thin sheet of quantum dots between two 2.5 mm thick sections of ex vivo chicken tissue. ( b – d ) Fluorescence emission camera images of the area (in the y – z plane) indicated by the dashed blue square in a . ( b ) Diffuse illumination pattern obtained by focusing into the tissue without wavefront modulation (flat phase display on the SLM). ( c ) Illumination pattern resulting from optical phase conjugation of ultrasound-tagged light, showing a focus on top of a diffuse background. ( d – f ) Background images and ( g – i ) corresponding background subtracted maps (positive values) obtained by the following techniques: ( d , g ) mechanically shifting the sample by 5 μm to disrupt phase conjugation; ( d , h ) digitally shifting the phase map by 50 pixels; and ( f , i ) modulating the original phase map by subdividing it into 8×16 areas and alternately adding 0 or π phase shift to each area (see Methods ). Scale bar, 500 μm. Full size image Background subtraction As discussed above, the diffuse background seen in Fig. 2c was expected because of the lack of complete control of the entire light field in a phase conjugation experiment. We further observed that the diffuse background was concentrated around the focus, an effect that was also reported by Vellekoop et al . when focusing light through a layer of highly scattering zinc oxide particles [28] . With a large number of speckles in the focus (see above), the presence of this background drastically reduced the contrast at the focus and poses a critical challenge to optical focusing using time reversal. With the DOPC system, however, the ability to digitally manipulate the phase conjugate field allows for the possibility of playing back a light field that closely mimics the background, thus enabling background subtraction. Accurate background subtraction requires better understanding of the cause of its spatial localization. One possible explanation of this effect is that it is caused by correlations in the scattering transmission matrix [28] . Thus, like the fidelity of the optical phase conjugate focus, the presence of a concentrated background would depend on the precise alignment of the sample with the phase-conjugated beam. Alternatively, the observed background could be caused by the macroscopic concentration of diffuse light around the target area—an effect that would be expected to be more prominent in highly forward-scattering samples such as biological tissues, and that would be invariant to microscopic misalignments of the sample. To identify the dominant effect contributing to the background in our forward-scattering sample, we displaced the sample by 5 μm and displayed the conjugate of the phase map recorded before the displacement. As can be seen in Fig. 2d , this shift entirely disrupted the focused beam, whereas the diffuse background was unaffected. After subtraction of this background from the raw image, a focus was revealed at much higher contrast ( Fig. 2g ). However, mechanical displacement is an impractical method for background subtraction for most applications. Instead, we can digitally alter the recorded phase maps to mimic the diffuse background illumination. We achieved this by two methods: digitally shifting the phase map by 50 pixels ( Fig. 2e,h ) or dividing phase maps into large subregions and phase-shifting every other subregion by π ( Fig. 2f,i ; see Methods )—a strategy related to differential background rejection techniques previously used in two-photon microscopy [39] , [40] . As digital shifting may introduce undesirable asymmetry to the phase map, the latter method for background subtraction was chosen for all subsequent experiments. We note that a suitable background image could not be obtained by simply displaying a flat phase map on the SLM (as shown in Fig. 2b ). Such approach would fail to adapt to different locations of the ultrasound focus and would be unable to compensate for geometrical aberrations in the tissue. Performing time reversal and subtracting the background in this manner for each location of the focus, we scanned the position of the ultrasound transducer and confirmed that the optical focus followed the locations of the ultrasound focus ( Supplementary Movie 1 ). Determining the point spread function To measure the point spread function and to quantify the resolution of our imaging system, we placed a fluorescent quantum dot filled polyacrylamide (PAA) bead (<20 μm in diameter) between two pieces of ex vivo chicken breast tissue ( Fig. 3a ). 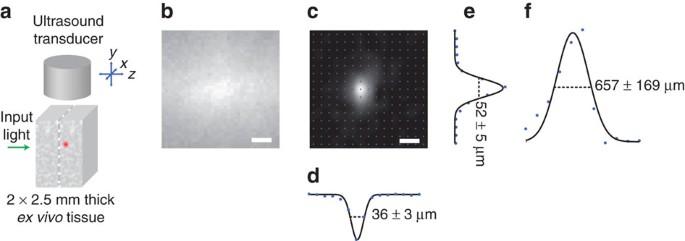Figure 3: Determination of point spread function. (a) Schematic of the setup used for the point spread function measurement. A fluorescent bead is embedded between two 2.5 mm thick sections ofex vivotissue. (b) Epifluorescence image of the sample in thexyplane, showing very strong blurring due to tissue scattering. (c) Fluorescence image obtained by scanning the position of the ultrasound transducer inxandy, detecting the fluorescence excited by time-reversed light and using adaptive background cancellation as described in the text. (d–f) Profile of the fluorescent bead inx(d),y(e) andz(f) direction. Blue dots indicate locations of collected data points. Pixels between data points are interpolated for display using bicubic interpolation. Scale bar, 50 μm. Figure 3b shows an epifluorescence image of this sample. Because of the forward scattering nature of our biological sample ( g =0.965; ref. 40 , 41 ), the approximate location of the bead can be inferred. However, tissue scattering results in very strong blurring that would prohibit imaging at high resolution. In contrast, Fig. 3c shows a well-resolved image of the bead collected using time-reversed light. To obtain the image, the ultrasound focus was scanned in the xy plane and an optical focus obtained by phase conjugation was formed at each scan position indicated by the blue dots. Background subtraction by dynamic digital phase map manipulation was performed at every step. As the bead is smaller than the ultrasound focus, the imaged size of the bead effectively estimates the three-dimensional resolution of the imaging system. The profiles in each dimension ( Fig. 3d–f corresponding to the x , y and z dimensions, respectively) were fit by Gaussian point spread functions with widths of 36±3 μm and 56±5 μm (full-width at half-maximum) in the plane perpendicular to the axis of light propagation, and 657±169 μm along the axis of light propagation (values ±95% confidence of fit). Figure 3: Determination of point spread function. ( a ) Schematic of the setup used for the point spread function measurement. A fluorescent bead is embedded between two 2.5 mm thick sections of ex vivo tissue. ( b ) Epifluorescence image of the sample in the xy plane, showing very strong blurring due to tissue scattering. ( c ) Fluorescence image obtained by scanning the position of the ultrasound transducer in x and y , detecting the fluorescence excited by time-reversed light and using adaptive background cancellation as described in the text. ( d – f ) Profile of the fluorescent bead in x ( d ), y ( e ) and z ( f ) direction. Blue dots indicate locations of collected data points. Pixels between data points are interpolated for display using bicubic interpolation. Scale bar, 50 μm. Full size image Fluorescence image of complex objects embedded in tissue We demonstrate the deep-tissue imaging capability of our system by raster scanning a known complex feature. We patterned quantum dot features of an abstract 'CIT' design in a 500-μm thin patch of PAA gel (a hydrogel that is commonly used for ultrasound phantoms [42] ), embedded between two pieces of chicken tissue, each 2.5 mm thick ( Fig. 4a ). 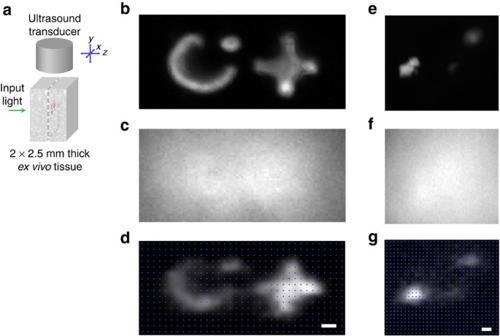Figure 4: Fluorescence image of complex objects. (a) Diagram of sample arrangement. (b) Epifluorescence image of an abstract 'CIT' feature. (c) Epifluorescence image obtained when the sample is placed under 2.5 mm of biological tissue. The features are not resolved. (d) Raster-scanned image of the embedded 'CIT' feature obtained using our imaging system. (e) Epifluorescence image of tumour microtissues. (f) Epifluorescence image obtained when the sample is placed under 2.5 mm of biological tissue. (g) Raster-scanned image of the embedded tumours obtained using our imaging system. Blue dots indicate locations of collected data points. Pixels between data points are interpolated for display using bicubic interpolation. Scale bars, 50 μm. Figure 4b shows an epifluorescence image of the features before embedding. Because of the tissue scattering, the embedded features cannot be resolved with epifluorescence imaging ( Fig. 4c ). In comparison, the 'CIT' features are clearly resolved using our method ( Fig. 4d ). Figure 4: Fluorescence image of complex objects. ( a ) Diagram of sample arrangement. ( b ) Epifluorescence image of an abstract 'CIT' feature. ( c ) Epifluorescence image obtained when the sample is placed under 2.5 mm of biological tissue. The features are not resolved. ( d ) Raster-scanned image of the embedded 'CIT' feature obtained using our imaging system. ( e ) Epifluorescence image of tumour microtissues. ( f ) Epifluorescence image obtained when the sample is placed under 2.5 mm of biological tissue. ( g ) Raster-scanned image of the embedded tumours obtained using our imaging system. Blue dots indicate locations of collected data points. Pixels between data points are interpolated for display using bicubic interpolation. Scale bars, 50 μm. Full size image Fluorescence image of embedded tumour microtissues We also obtained images of tumour microtissues embedded in tissues. The microtissues are arranged in a 500-μm thin patch of PAA gel, embedded between two pieces of chicken tissue, each 2.5 mm thick. Figure 4e shows an epifluorescence image of the tumours. The tumours embedded between ex vivo tissue are not resolved with epifluorescence imaging ( Fig. 4f ). In contrast, the tumours imaged with our method are well resolved and the differential fluorescence intensities of the tumours are also reflected in the image ( Fig. 4g ). Fluorescence imaging in biological tissues beyond one transport mean free path is one of the most challenging goals in biomedical optics. In this study, we provide the first demonstration of focal fluorescence imaging in the diffusive regime with time reversal of ultrasound-tagged light. We implemented a DOPC system with high gain to directly observe the time-reversed optical focus and the accompanying phase conjugate background. We took advantage of the capabilities of the DOPC to digitally manipulate the phase-conjugate map to dynamically estimate and subtract the fluorescence contribution of the phase conjugate background that would otherwise obscure the focal fluorescence signal. Using this technique, we characterized the point spread function of the system as having an anisotropic lateral resolution of 34 μm×52 μm and an axial resolution of 657 μm. Furthermore, we illustrated the capabilities of our method by successfully imaging fluorescent objects 2.5 mm deep in ex vivo tissue, equivalent to about 75 scattering mean free paths [30] . As confirmed by our results, the imaging resolution perpendicular to the axis of light propagation is determined by the ultrasound focal volume. The system's resolution can therefore be improved by using an ultrasound transducer with a higher central frequency and a higher numerical aperture. However, some expected tradeoffs should be noted. Higher frequency ultrasound is more strongly attenuated in biological tissues [43] , thus reducing the practical focusing depth of the ultrasound. In addition, a smaller modulation volume would further diminish the population of the frequency-shifted light and increase the challenge of detecting a small signal on top of a large background during phase measurement. However, these issues can be addressed by the development of faster, higher dynamic-range cameras, and with advanced filtering methods [44] , [45] . The point spread function along the axis of light propagation is limited by the angular spread of the focused light cone. As the angular spread is a function of illumination geometry and tissue scattering, the resolution could be improved by using high-numerical aperture illumination or—counter-intuitively—by imaging thicker, more scattering samples. Finally, the resolution along the axis of light propagation could further be improved by taking advantage of multiphoton excitation. We estimate that at the plane of the time-reversed focus, <1% of the energy is within the focus. This means that ~99% of the remaining energy is spread over the diffuse background, which if uncorrected can obscure the focal fluorescence signal. In non-homogeneous fluorescent samples, we showed that dynamic background subtraction effectively uncouples the focal fluorescence signal from that excited by the background. In some applications like photodynamic therapy, where the goal is to deliver more light into the focus, a further increase in peak-to-background ratio may be desirable. There are two ways to achieve a higher peak-to-background ratio. First, the number of optical modes ( N ) controlled by the DOPC can be increased by increasing the number of pixels on the SLM. Second, the number of optical modes in the ultrasound focus ( M ) can be decreased by decreasing the size of the ultrasound focus. Because our method is based on optical time reversal, it relies on mechanical stability of the sample. The acquisition cycle per pixel should therefore be faster or on the same order of magnitude as the speckle decorrelation of the tissue. This condition is easily met in ex vivo experiments: our current pixel acquisition time (6.7 s) was shorter than the decorrelation time of the sample (41 s). For in vivo applications, decorrelation times are typically much faster: published values range from the order of milliseconds [46] , [47] , [48] to seconds [49] , depending on the tissue type and immobilization strategies. For such applications, the pixel acquisition time would have to be reduced accordingly. We anticipate that this will ultimately be possible with the use of faster SLMs [50] , and with the continuing development of faster, higher dynamic range cameras. In all our experiments, the irradiance of the laser beam at the sample was <10 mW mm −2 . The laser power would have to be decreased, or the diameter of the beam increased, to meet clinical safety standards (2 mW mm −2 ). Taken together, such improvements would ultimately enable a wide range of in vivo applications, including molecular imaging, early cancer diagnosis, photodynamic therapy and targeted excitation of optogenetic tools in deep tissues. Sample preparation Frozen ex vivo chicken breast tissue was cut into 2.5 mm thick slices and embedded in 10% PAA gel inside an open-top quartz glass sample cuvette with four polished sides (Starna Cells, CA). The tissue slices had a measured scattering coefficient of μ s =30 mm −1 (see also ref. 30 ). Using the previously published anisotropy [41] of g =0.965, we calculated the reduced scattering coefficient to be μ ′ s = μ s (1− g )=30 mm −1 · (1−0.965)=1.05 mm −1 . This is in agreement with the widely referenced approximate value of ~1 mm −1 (see for example, refs 5 , 20 ). The PAA gel was polymerized using 4 ml phosphate-buffered saline, 1.5 ml acrylamide, 0.4 ml bis-acrylamide, 62.5 μl ammonium persulfate and 25 μl tetramethylethylenediamine. PAA beads containing quantum dots (Qtracker 655 Non-targeted Quantum Dots, Invitrogen) were made using a reverse micelle protocol modified from Beningo and Wang [51] with a starting concentration of 200 nM quantum dots in the aqueous phase. The beads obtained varied in size and were strained through a 40 μm cell strainer (Biologix, USA). The actual sizes of the beads used in all experiments were determined by observation under a fluorescence microscope. The 'CIT' feature was made by polymerizing clear PAA gel (500 μm thick) on a SU-8 mold (designed in-house, manufactured by the Stanford Microfluidics Foundry). The patterned depression in the clear PAA gel was then filled with PAA containing quantum dots (Qtracker 705 Non-targeted Quantum Dots, Invitrogen) with a starting concentration of 1 μM in the aqueous phase. Cancer microtissues, obtained by the hanging-drop technique using HepG2 cells [52] , were custom ordered from InSphero AG (Switzerland). The spheroids were fixed with 2% paraformaldehyde (Sigma-Aldrich, USA), washed with 50 mM borate buffer saline (Thermo Scientific, USA), permeabilized with 0.1% Triton-X 100 (Sigma-Aldrich, USA), and stained with DY-521XL long stokes shift NHS-ester dye (Dyomics, Germany) that binds to the proteins in the cancer microtissues. The concentration of the staining solution was 14 nM. Based on calibration with known fluorophore concentrations, we estimated the resulting stain concentration in the tumour to be ~5 μM. The tumour microtissues were arranged and embedded in a 500-μm thin PAA gel patch. Measurement of sample scattering coefficient The scattering coefficient of the chicken tissue was measured interferometrically with a Mach–Zehnder interferometer. As only ballistic light significantly interferes with the reference beam, the reduction in amplitude of the fringes with and without a sample in the sample beam path could be used to find the scattering coefficient [30] . Setup All data shown was recorded using a custom-built experimental setup diagrammatically shown in Supplementary Fig. S1 . A 2.7 W, 532 nm Q-switched laser (Navigator, SpectraPhysics, USA) pulsed at 20 kHz with a pulse width of 7 ns and a coherence length of 7 mm was used as a light source at optical frequency f 0 . After passing an optical isolator and a fixed attenuator, it was split into a reference beam and a sample beam. The sample beam was attenuated by a neutral density filter wheel, spatially filtered by a single mode optical fibre (Nufern 460HP, 20 cm length), collimated to a 0.8-mm waist beam and directed into the sample cuvette. The irradiance at the sample was ~10 mW mm −2 . We note that this is above the ANSI standards for skin irradiance (2 mW mm −2 ). However, we do not foresee lowering the laser power as being a fundamental limitation. Inside the sample, a fraction of the light was frequency-shifted to f 0 + f US by an ultrasound transducer (element size: 6.35 mm, focal length: 6 mm; V3330, Olympus NDT, Olympus, USA) operated at f US =45 MHz. To achieve maximal resolution along the axis of ultrasound propagation, the transducer was driven with short pulses (pulse length: 1 cycle at 45 MHz, 55 V peak-to-peak) triggered by the laser Q-switch signal at a fixed delay such that the ultrasound pulses coincided with the laser pulses at the ultrasound focus [32] (the trigger delay was jittered by ±5.5 ns to minimize the detection of coherent effects between ultrasound-tagged and untagged light; see Supplementary Methods ). To scan the ultrasound focus, the transducer was mounted on a three-axis computer-controlled micromanipulator (Sutter Instruments, USA). After passing through the sample, the scattered beam was recombined with the reference beam (horizontally-polarized), which had also been frequency-shifted by f US by an acousto-optic modulator (AFM-502-A1, IntraAction, USA). After passing a horizontally-aligned polarizer and another beamsplitter, the combined beams reached the surface of a phase-only SLM (vis-PLUTO, Holoeye, Germany), carefully aligned (1:1 pixel-to-pixel match) to the image plane of a high dynamic range sCMOS camera (pco.edge, PCO AG, Germany). The lens used to image the SLM onto the sCMOS camera was a commercial compound lens (Micro-Nikkor 105 mm f/2.8, Nikon). Compared with the DOPC system first described by Cui and Yang [31] , our improved DOPC system directly imaged the SLM pixels onto the camera pixels, and thus, enabled reliable alignment and day-to-day quality assurance (see below). As the image had to be reflected by a beamsplitter, we chose a plate beamsplitter (High-Energy Nd:YAG 50/50, Newport Corporation, CA) whose reflective surface faced both the SLM and the camera, so as to avoid image aberrations and ensure precise alignment. SLM curvature compensation The reliability of DOPC critically depends not only on the precise alignment of the SLM and the camera, but also on the SLM curvature and the reference beam aberrations. Both of these effects can be compensated for digitally by finding a compensation phase map for the SLM that, when displayed, time reverses the reference beam. Because a time-reversed beam would trace its path back through the spatial filter (the SM fibre), the compensation map was optimized by maximizing the power of the light that returned back through the single-mode fibre (measured by a photodiode). Phase recording At each scan position, phase recording was achieved in a phase-shifting digital holography setup [36] : the ultrasound pulse was cycled through four phases (0, π/2, π, 3π/2). A total of 10–30 frames were recorded (at 30 frames per second) for each phase and averaged, resulting in four intensity maps ( I 0 , I π/2 , I π and I 3π/2 ), which were used to reconstruct the complex field according to E =( I π/2 − I 3π/2 )+ i ( I 0 − I π ). The phase map was calculated as Φ =tan −1 (Re( E )/Im( E )) (or Φ=Arg( E )). To minimize artifacts introduced by slow phase fluctuations of the reference beam, the acquisition of the intensity maps was interleaved by cycling through all four phases for each block of four sequential frames acquired by the sCMOS camera (exposure time: 28 ms, frame rate: 30 Hz). To achieve sufficiently fast cycling and between-frame switching, an arbitrary function generator (AFG 3252, Tektronix, USA) generated two output signals (one 45 MHz sinusoidal cycle with phase shift of 0 or π/2), which were each inverted by an RF 180° power splitter (Mini-circuits, USA) to obtain the four phase-shifted signals. A microcontroller board (Arduino, Italy; obtained from SparkFun Electronics, USA) connected to an RF switch (Mini-circuits, USA) was programmed to select the appropriate phase for each frame acquired by the sCMOS camera. Throughout the phase recording, the SLM displayed a flat (all 0) phase map. An acquisition cycle took 6.7 s per pixel. For complete timing information, see Supplementary Fig. S2 . For an analysis of whether the coherence length limits detection of scattered photons, see Supplementary Fig. S3 . A typical ultrasound-tagged phase map recorded on the camera contained N =8×10 4 modes (area of the sensor divided by speckle autocorrelation area). Together with an estimated M (number of speckles in the ultrasound focus) of 1–2×10 3 we obtained an upper bound for the peak-to-background ratio of ~60 (equation (3)). Detection of fluorescence excitation by time-reversed light The time-reversed beam was obtained by reflecting the blank reference beam off the SLM displaying the measured phase conjugate map. The backscattered fluorescence excited by the time-reversed optical focus was reflected off a dichroic mirror and detected by a single-channel PMT fitted with the appropriate bandpass filters (Semrock 650-40, 710-40 or 675-67, for Qtracker 655, Qtracker 705 or DY-521XL long stokes shift NHS-ester dye, respectively). Quality assurance of DOPC Because of the dependence of our system on precise alignment, mechanical stability and low drift, we included a parallel sample beam path to assess and assure the performance of our setup on a day-to-day basis. Consisting of ground glass diffusers and an additional observing camera, it was analogous to the setups previously used by our group to demonstrate turbidity suppression by phase conjugation [30] . Speckle decorrelation time With the sample beam turned on, we acquired images of the speckle field on the sCMOS camera at a rate of 1 frame per second for 180 s. We measured the correlation of the first frame with each subsequent frame and defined the decorrelation time as the time after which the correlation fell below 1 − 1 / e . How to cite this article: Wang, Y. M. et al . Deep-tissue focal fluorescence imaging with digitally time-reversed ultrasound-encoded light. Nat. Commun. 3:928 doi: 10.1038/ncomms1925 (2012).